Magnetochiral dichroism resonant with electromagnons in a helimagnet Cross-coupling between magnetism and electricity in a solid can be hosted by multiferroics with both magnetic and ferroelectric orders. In multiferroics, the collective spin excitations active for both electric and magnetic fields, termed electromagnons, play a crucial role in the elementary process of magnetoelectric (ME) coupling. Here we report the colossal dynamical (optical) ME effect, or more specifically the magnetochiral (MCh) effect, in the electromagnon resonance for the screw spin helimagnet CuFe 1− x Ga x O 2 ( x =0.035). The MCh effect shows up as the nonreciprocal directional dichroism; the extinction coefficient is different for counter-propagating lights, as large as by 400%. The MCh effect derived from the screw spin order is proved by control of the magnetic helicity of helimagnetism and its magnetization. The results point to the general presence of the MCh effect in helimagnets, paving a way to the ME control of electromagnetic wave in the giga- to tera-hertz region. The magnetoelectric (ME) effect, in which electric polarization and magnetization in a matter are respectively controlled by magnetic and electric fields, has been attracting renewed attention for its possible applications to spintronics and magneto-optical devices [1] , [2] , [3] . Inherently strong ME effects have been found in the multiferroics whose ferroelectricity is induced by particular spin structures [4] , [5] , [6] . Among them, one unique mechanism for multiferroicity of spin origin is the spin–current model [7] or inverse Dzyaloshinskii–Moriya interaction [8] , [9] ; the ferroelectric polarization ( P ) is induced by the spin supercurrent flowing between the mutually canted neighbouring spins ( S i and S j ) under the presence of relativistic spin–orbit interaction and expressed as P ∝ e ij × ( S i × S j ), where e ij denotes the unit vector connecting the neighbouring spin sites. According to this mechanism, a cycloidal (transverse helical) spin structure shows the macroscopic ferroelectric polarization ( P ), in which the helicity of the spins is responsible for the sign of P , that is, a change of the spin helicity coincides with a reversal of the P , whereas the screw (longitudinal helical) structure cannot induce the ferroelectricity by the spin–current mechanism. A fluctuation of the multiferroic spin order produces a concomitant novel spin excitation, termed electromagnon, which is an electrically dipole active spin wave excitation [10] , [11] , [12] , [13] , [14] , [15] . One important outcome of the electromagnon excitation is to mediate the dynamical (optical) ME effect; the resonance is ME in nature, that is, responding to both a.c. (optical) electric and magnetic fields [14] , [15] , [16] , [17] , [18] . This cross-coupled response to light leads to the novel optical property termed directional dichroism, which differentiates the optical responses for two counter-propagating light beams [19] , [20] . Such an optical ME effect is based not only on the electric activity but also the magnetic activity of the electromagnon resonance. Among the electromagnons, the spin–current mechanism can host a strong optical ME effect, because the spin-driven character of ferroelectric polarization enables the coupling between the simultaneous fluctuation of uniform magnetization and electric polarization on the electromagnon resonance. In fact, the conspicuous optical ME effect with the electromagnon in the (conical) cycloidal magnet, which simultaneously satisfies the symmetrical condition for the occurrence of the optical ME effect, has been observed [14] , [15] . Since the optical ME effect is allowed under the simultaneous breaking of the time-reversal and the space-inversion symmetries, the multiferroicity gives rise to the optical ME effect. In the conical cycloidal magnet, both P and M are derived from the spin order, so that the fluctuations of ferroelectric polarization ( ΔP ω ) and magnetization ( ΔM ω ) are strongly coupled with each other as a dynamical counterpart of the multiferroicity at the ground state, leading to the gigantic optical ME effect [14] , [15] , [21] . On the other hand, another route to the optical ME effect can be provided by the coexistence of the lattice or electronic chirality and the magnetization, which is called magnetochiral (MCh) effect [19] , [20] , [21] , [22] , [23] , leading to the directional dichroism for the lights propagating parallel and antiparallel to the magnetization. The chirality is represented by two inequivalent mirror images such as clockwise helix and counter-clockwise helix. (Hereafter, we denote them as γ m (+) and γ m (−).) Accordingly, a helix derived from spin texture, that is, screw spin structure ( Fig. 1a ), provides the matter with chirality irrespective of the symmetry of the underlying lattice system, or even in achiral (or centrosymmetric) lattice structure at the paramagnetic state. Because the conical screw spin structure ( Fig. 1a ) also produces the net magnetization as well as the chirality, the necessary conditions of the MCh effect are satisfied exclusively by such a spin structure. The MCh effect for the electromagnon resonance has been theoretically predicted based on the spin–current mechanism [21] . As shown in the Fig. 1a , the uniform fluctuation of the cone axis of the conical screw spins, which induces a fluctuation of the magnetization ( ΔM ω ), generates the transient cycloidal spin component, leading to the uniform polarization ( ΔP ω ) perpendicular to the ΔM ω , irrespective of presence or absence of static P . Both ΔM ω and ΔP ω interact with the magnetic field ( H ω ) and electric field ( E ω ) of the light, respectively, so that the optical response depends on the direction of the light ( k ω ). As an important feature of the MCh effect, the reversal of the directional dichroism is also caused by the reversal of either chirality ( γ m ) or magnetization ( M ). In the conical screw structure, the change of chirality (or spin helicity) reverses the direction of ΔP ω , resulting in the sign change of the MCh effect (see γ m (+) and γ m (−) in Fig. 1a ). This character explicitly distinguishes the MCh effect from the magneto-circular dichroism or Faraday rotation effect, which is always expected more or less in this optical geometry. 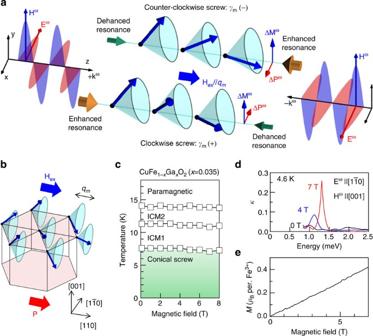Figure 1:  Magnetochiral dichroism in a helimagnet and magnetic properties of CuFe1−xGaxO2forx=0.035. (a) Schematics of MCh dichroism for a helimagnet with conical screw spin structure. Single helicity domain (clockwise or counter-clockwise screw) is prepared and d.c. magnetic field (Hex) renders conical screw spin structure. Wave vector of the incident light (±kω) is parallel or antiparallel to the magnetic modulation vector (qm), that is, ±kω//Hex//qm. The induced magnetization (ΔMω) by light simultaneously produces a dynamical electric polarization (ΔPω) via the spin–current mechanism21,33. (See text for details.) The responses ofΔMωandΔPωto the magnetic field (Hω) and electric field (Eω) of light differentiate absorption between oppositely propagating light beams (+kωor−kω), namely, directional dichroism occurs, as indicated by ‘enhanced resonance’ and ‘dehanced resonance’. (The relative direction betweenEωandHω, which changes with the sign ofkω, shows in-phase or out-of-phase correspondence for the interlockedΔMωandΔPω.) The change of the chirality (or spin helicity) described as clockwise screwγm(+) or counter-clockwise screwγm(−) also reverses the interlocked dynamical polarization (ΔPω), resulting in the reversal of the directional dichroism. (b) The conical screw spin structure under external magnetic field (Hex). The external magnetic field (Hex) parallel to the in-plane magnetic modulationqm(for example, // [110]) modifies the proper screw spin structure to the conical one. The ferroelectric polarization (P) driven by the screw spin structure viad–porbital hybridization mechanism (see text) also points to the in-planeqmdirection ([110]). (c) Magnetic phase diagram under magnetic field (Hex|| [110]). Frustration of the Fe3+spins leads to the successive magnetic phase transitions from a paramagnetic phase to two incommensurate collinear (ICM) spin phases and to the conical screw spin phase. (d) Imaginary part of the refractive indexκ(ω) for the light polarized alongEω|| [001],Hω|| [10] under the magnetic field (Hex||[110]). (e) Magnetization curve under the magnetic field parallel to [110] axis29. Figure 1:  Magnetochiral dichroism in a helimagnet and magnetic properties of CuFe 1 −x Ga x O 2 for x =0.035. ( a ) Schematics of MCh dichroism for a helimagnet with conical screw spin structure. Single helicity domain (clockwise or counter-clockwise screw) is prepared and d.c. magnetic field ( H ex ) renders conical screw spin structure. Wave vector of the incident light (± k ω ) is parallel or antiparallel to the magnetic modulation vector ( q m ), that is, ± k ω // H ex // q m . The induced magnetization ( ΔM ω ) by light simultaneously produces a dynamical electric polarization ( ΔP ω ) via the spin–current mechanism [21] , [33] . (See text for details.) The responses of ΔM ω and ΔP ω to the magnetic field ( H ω ) and electric field ( E ω ) of light differentiate absorption between oppositely propagating light beams (+ k ω or− k ω ), namely, directional dichroism occurs, as indicated by ‘enhanced resonance’ and ‘dehanced resonance’. (The relative direction between E ω and H ω , which changes with the sign of k ω , shows in-phase or out-of-phase correspondence for the interlocked ΔM ω and ΔP ω .) The change of the chirality (or spin helicity) described as clockwise screw γ m (+) or counter-clockwise screw γ m (−) also reverses the interlocked dynamical polarization ( ΔP ω ), resulting in the reversal of the directional dichroism. ( b ) The conical screw spin structure under external magnetic field ( H ex ). The external magnetic field ( H ex ) parallel to the in-plane magnetic modulation q m (for example, // [110]) modifies the proper screw spin structure to the conical one. The ferroelectric polarization ( P ) driven by the screw spin structure via d – p orbital hybridization mechanism (see text) also points to the in-plane q m direction ([110]). ( c ) Magnetic phase diagram under magnetic field ( H ex || [110]). Frustration of the Fe 3+ spins leads to the successive magnetic phase transitions from a paramagnetic phase to two incommensurate collinear (ICM) spin phases and to the conical screw spin phase. ( d ) Imaginary part of the refractive index κ ( ω ) for the light polarized along E ω || [001], H ω || [10] under the magnetic field ( H ex ||[110]). ( e ) Magnetization curve under the magnetic field parallel to [110] axis [29] . Full size image Here we demonstrate a gigantic MCh effect in resonance with electromagnon in the helical spin structure for delafossite CuFe 1 −x Ga x O 2 ( x =0.035) by the terahertz time-domain spectroscopy. For the electromagnon resonance at 1.3 meV, the presence of the MCh effect is confirmed under the control of the magnetization as well as the spin helicity ( γ m ). The observed directional dichroism possesses the high contrast in the extinction coefficient κ ( ω ) up to 400%, manifesting the inherent strong ME cross-coupling of the helical magnet. Magnetism and magnetic resonance in a helimagnet The MCh effect on the electromagnon resonance for the screw spin structure is demonstrated on the delafossite-type copper iron oxide CuFe 1 −x Ga x O 2 ( x =0.035). The competition of the exchange interactions as well as the geometrical frustration among the Fe 3+ spins ( S =5/2) in the triangular-lattice plane ( Fig. 1b ), which stacks along [001] direction, results in the complex magnetic phase diagram including the screw spin structure [24] , [25] . The slight doping of the non-magnetic ions, such as the Al [26] , [27] and Ga [28] , [29] , stabilizes the screw spin phase, whose magnetic modulation vector has an incommensurate wave number (q, q, 3/2) with q =0.202 below 7.4 K (see Fig. 1b,c ). Hereafter, we simplify the magnetic modulation vector q by extracting the in-plane component; q =(q, q, 0). There are three equivalent [110] axes for the in-plane direction as well as the helicity degree of freedom of the screw spins, that is, clockwise or counter-clockwise, resulting in sixfold degeneracy in the screw spin state under zero magnetic field. To corroborate the MCh effect driven by the screw spin structure, the single q - and single chiral ( γ m )-domain is indispensable. In this compound, ferroelectricity has been observed in the screw spin phase, where the hybridization of the metal (Fe 3+ ) d state and ligand (O 2− ) p state under the influence of spin–orbit interaction ( d–p orbital hybridization model) has been suggested as the origin of the ME coupling [30] , [31] , whereas the spin–current mechanism cannot contribute to the presence of the P in this screw spin phase, since e ij × ( S i × S j )=0. The ferroelectric polarization ( P ) appears parallel to the magnetic q vector, and the helicity of the screw spin structure is responsible for the sign of P . Accordingly, a ME-cooling process enables us to manipulate the helicity- and q -domains. Detail of the manipulation process is described in the Methods section. The optically active spin wave excitation has been measured for the single-domain conical screw spin state ( Fig. 1d ). The propagation vector of light ( k ω ), the external magnetic field ( H ex ) and the magnetic modulation vector q are parallel with each other, that is, in Faraday geometry ( Fig. 1a ). The characteristic excitation mode in the conical screw spin structure has been observed under the magnetic field as shown in Fig. 1d . This resonance can be ascribed to the fluctuation of the net magnetization, that is, uniform oscillation of the cones around q vector (see Fig. 1a ). In fact, the intensity develops with increasing the magnetization by external magnetic field H ex as shown in Fig. 1d,e . The ME features of this resonance are examined under the control of helicity and magnetization. Although the Faraday rotation inevitably affects the polarization of light in this geometry, the rotation angle is sufficiently small, allowing us to employ the quasi-linear polarization analysis below 7 T. (Note that the magnetization is <10% of the full moment of the Fe 3+ spins below 7 T as shown in Fig. 1e [29] ; see Methods for details.) MCh effect of screw spin structure The optical MCh effect showing the nonreciprocal directional dichroism for the linearly polarized light can be described by the ME term α for the complex refractive index as follows [21] , [32] , [33] . Under the coexistence of chirality and magnetization ( M ), which breaks the time-reversal and space-inversion symmetry, the first-order ME effect described by ME tensor is allowed. Then, the dynamical electric polarization ( P ω ) and magnetization ( M ω ) turn out to be a cross-coupled response to the electric ( E ω ) and magnetic ( H ω ) field of the light propagating parallel to M as follows. Here the α ij ( ω ) is an element of the ME tensor, and the χ ee and χ mm are the ordinary electric and magnetic susceptibilities, respectively. By combining the above relations with Maxwell’s equations on the assumption of the plane wave and linearly polarized light [33] , the wave vector of light turns out to have directional character; k ω z =± ω (( n 0 ( ω )+ i κ 0 ( ω ))+ ω α ij ( ω ). ( k ω z is assumed to be the nonzero component of k ω .) Accordingly the k ω -direction-dependent optical response is yielded due to the ME-coupling term α ij [33] . In addition to the ordinary term of the refractive index ( n 0 ( ω )+ iκ 0 ( ω )), the real and imaginary parts of α ij ( ω ) contribute to the optical response [21] . The sign of the directional dichroism (± α ij ( ω )) is determined by product of the signs of chirality ( γ m =±1), magnetization (± M ) and propagation vector (± k ω ), that is, (± k ω )·( γ m )·(± M ) [34] . The MCh dichroism was examined for the magnetic resonance excitation of the conical screw spin structure with single q - and helicity- domain in a single crystal of CuFe 1 −x Ga x O 2 ( x =0.035). 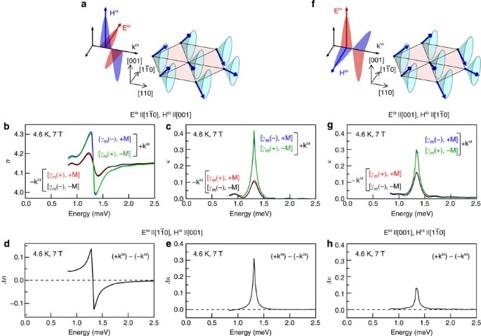Figure 2: Gigantic magnetochiral dichroism in the helimagnet. Schematic illustration for the light polarization configurations, (a)Eω|| [10],Hω||[001], and (f)Eω|| [001],Hω|| [10] for the conical screw spin structure on the delafossite (001) plane. The spectra of (c) real partn(ω) and (d) imaginary partκ(ω) of the complex refractive index at 4.6 K and 7 T (Hex|| [110]) with the light configuration ina. Spectra with both signs of spin helicity (γm=+or−) and magnetization (+Mor−M) are shown. Complex magnetoelectric (ME) spectra defined as (d) Δn(ω)=n(+kω)−n(−kω) and (e) Δκ(ω)=κ(+kω)−κ(−kω) derived frombandc, respectively. For the crossed light polarization inf, the imaginary part of (g) the refractive indexκ(ω) and (h) the ME spectra Δκ(ω) at 7 T (Hex|| [110]) are also displayed. Figure 2 shows the geometry for terahertz optical spectroscopy (a and f), extinction coefficient ( κ ( ω )) spectra (c and g) and ME spectra ( Δκ ( ω )) (e and h) as well as for the refractive indices ( n ( ω ) and Δn ( ω )) (b and d). When the electric field of light is parallel to the in-plane direction ( E ω ||[10], H ω ||[001]), the optical response remarkably changes with reversal of either the magnetization M or the sign of chirality γ m , being consistent with the character of the MCh effect (see Fig. 2b,c ). (Note that either operation is equivalent to the reversal of k ω direction while keeping M and γ m intact [34] .) Thus, the presence of the MCh effect is conclusively confirmed for this electromagnon resonance. The extinction coefficient with change of the experimental configuration changes from 0.1 to 0.4 due to the MCh directional dichroism, namely, 400% of the contrast in κ ( ω ) is observed for the resonance ( Fig. 2c ). Since the four possible states [ γ m (±), ± M ] in our experiments can be grouped into two inequivalent states in terms of the MCh configuration [34] , we denote them as ± k ω hereafter for the sake of simplicity (see Fig. 2b,c ). The difference of the extinction coefficient κ ( ω ) for + k ω and− k ω gives the ME spectra Δ κ ( ω )=Im [ N + ( ω )− N − ( ω )]=Im [2 α ij ( ω )] (see equation (2)) as shown in the Fig. 2e . The ME spectrum Δ κ ( ω ) shows the sharp resonance with the electromagnon excitation at 1.3 meV, whose peak is higher than 0.3. Figure 2: Gigantic magnetochiral dichroism in the helimagnet. Schematic illustration for the light polarization configurations, ( a ) E ω || [10], H ω ||[001], and ( f ) E ω || [001], H ω || [10] for the conical screw spin structure on the delafossite (001) plane. The spectra of ( c ) real part n ( ω ) and ( d ) imaginary part κ ( ω ) of the complex refractive index at 4.6 K and 7 T ( H ex || [110]) with the light configuration in a . Spectra with both signs of spin helicity ( γ m =+or−) and magnetization (+ M or− M ) are shown. Complex magnetoelectric (ME) spectra defined as ( d ) Δ n ( ω )= n (+ k ω )− n (− k ω ) and ( e ) Δκ(ω)=κ(+ k ω )−κ(− k ω ) derived from b and c , respectively. For the crossed light polarization in f , the imaginary part of ( g ) the refractive index κ ( ω ) and ( h ) the ME spectra Δ κ ( ω ) at 7 T ( H ex || [110]) are also displayed. Full size image For another light polarization, in which E ω is perpendicular to the in-plane direction ( E ω ||[001], H ω ||[10], see Fig. 2f ), the MCh dichroism is also confirmed as shown in the Fig. 2g . The sign of the directional dichroism is the same with the former configuration; the optical response for the + k ω has a higher resonance peak than for that for− k ω . This qualitatively isotropic ME response of the electromagnon is caused by the isotropic character of the screw spin structure within the plane normal to the magnetic q vector (// ± k ω ). The peak intensity of the ME resonance in Δ κ ( ω ) ( Fig. 2h ) is 0.14 at 1.3 meV, which is half of the former one. Although the fundamental behaviours are similar for both configurations, the highly anisotropic underlying chemical lattice character may differentiate the ME properties. Note that the static dielectric constants ε for E || [001] is as large as half of that for E ⊥ [001] [13] . The MCh dichroism has been examined across the successive magnetic transitions with elevating temperature at 7 T ( Fig. 3 and see the phase diagram in Fig. 1c . ). Within the temperature range below 6.5 K, that is, in the screw spin phase, the directional dichroism for the electromagnon spectra ( Fig. 3a ), as characterized by the ME spectra Δ κ ( ω ) ( Fig. 3b ), is clearly observed, while accompanying a slight softening of the resonance energy with the increase of temperature. In contrast, the sudden suppression of the directional dichroism is observed across the phase transition, for example, at 7.5 K, as shown in Fig. 3a,b . Although the magnetic resonance itself is discerned at 1.2 meV also in the incommensurate collinear spin phase 1 ( Fig. 3a ), the ME character (Δ κ ( ω )) of the mode clearly disappears. 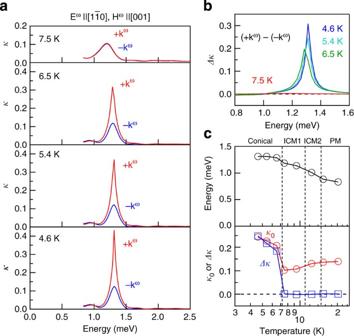Figure 3: Temperature dependence of magnetoelectric resonance. (a) Temperature dependence of the imaginary part of refractive indexκ(ω) at 7 T (Hex|| [110]) for two possible ME configurations denoted by +kωand−kω. (b) Temperature dependence of the ME spectra (Δκ(ω)) derived froma. (c) Temperature dependence of the resonance energy (upper panel), peak intensities of the normal termκ0(ω)=(κ(+kω)+κ(−kω))/2 and the ME term Δκ(lower panel) (see text for details). Figure 3: Temperature dependence of magnetoelectric resonance. ( a ) Temperature dependence of the imaginary part of refractive index κ ( ω ) at 7 T ( H ex || [110]) for two possible ME configurations denoted by + k ω and− k ω . ( b ) Temperature dependence of the ME spectra (Δ κ ( ω )) derived from a . ( c ) Temperature dependence of the resonance energy (upper panel), peak intensities of the normal term κ 0 ( ω )=( κ (+ k ω )+ κ (− k ω ))/2 and the ME term Δ κ (lower panel) (see text for details). Full size image The temperature dependence of the peak energy and intensity for normal term κ 0 as well as for ME term (Δ κ ( ω )) is plotted in the Fig. 3c . While the resonance energy monotonously decreases with increasing temperature, the intensity of the ME resonance (Δ κ ( ω )) drops abruptly to zero upon the transition from screw spin phase to the incommensurate collinear spin phase 1. Therefore, these results manifest that the screw spin structure or helicity of them are indispensable for the MCh effect, as expected. The step-like reduction of the normal term κ 0 ( ω ) upon the phase transition is ascribed perhaps to the loss of the electrical activity (electromagnon nature) in the magnetic resonance. The magnetic field dependence shown in Fig. 4 can unveil the ME character of the electromagnon resonance. With increasing magnetic field, the electromagnon resonance increases in intensity as well as the magnitude of their directional dichroism ( Fig. 4a,b ). The peak energy and intensities of ordinary term κ 0 ( ω ) and ME term Δ κ ( ω ) are plotted in Fig. 4c . The resonance energy increases from 1.0 meV at 1 T to 1.3 meV at 7 T, indicating that the external magnetic field stabilizes the screw spin state. The ME resonance Δ κ ( ω ) (blue square) monotonically increases with increasing the magnetic field or magnetization (see also Fig. 1e ), because the ME effect is proportional to the M around M =0. 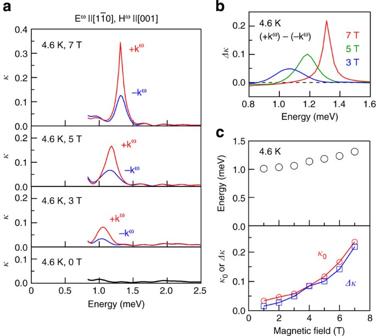Figure 4: Magnetic-field dependence of magnetoelectric resonance. (a) Spectra of the imaginary part of the refractive indexκ(ω) under the magnetic field along [110] for two distinct ME configurations denoted by +kωand−kω. (b) Magnetic-field dependence of the ME spectra (Δκ(ω)) derived froma. (c) Magnetic-field dependence of the resonance energy (upper panel), peak intensities of the normal termκ0(ω)=(κ(+kω)+κ(−kω))/2 and the ME term Δκ(lower panel) (see text for details). Figure 4: Magnetic-field dependence of magnetoelectric resonance. ( a ) Spectra of the imaginary part of the refractive index κ ( ω ) under the magnetic field along [110] for two distinct ME configurations denoted by + k ω and− k ω . ( b ) Magnetic-field dependence of the ME spectra (Δ κ ( ω )) derived from a . ( c ) Magnetic-field dependence of the resonance energy (upper panel), peak intensities of the normal term κ 0 ( ω )=( κ (+ k ω )+ κ (− k ω ))/2 and the ME term Δ κ (lower panel) (see text for details). Full size image We have so far postulated the spin–current mechanism as an origin of the MCh dichroism resonant with the electromagnon [7] , [21] , [33] . As an alternative origin, one may consider the possibility that the P driven by the d – p orbital hybridization mechanism is involved in the generation process of the electromagnon [30] , [31] , namely that the fluctuation of P can give the electrical activity to the excitation of the screw spin structure, as scaled by P 2 according to the fluctuation-dissipation theorem. As shown in the Fig. 4a,c , the electromagnon resonance clearly develops under the magnetic field, while the peak structure is hardly distinguishable at 0 T. In this compound, the ferroelectric polarization P is almost intact under the magnetic field (<7 T) [29] . Accordingly, apparent discrepancy of the electromagnon intensity from P 2 indicates that the fluctuation of spontaneous P is almost irrelevant to the presently observed electromagnon excitation. Among the several dichroic optical effects, such as magneto-circular dichroism, natural optical activity and optical ME effects, the MCh effect is a latecomer, which has been discovered in 1997 (ref. 22) [22] . In most cases including the optical or X-ray region, the dichroic character arises from the local atomic environment [35] , [36] , while this electromagnon reflects the long-range order of spins. In fact, MCh effect has been reported for electronic transitions in the visible [22] , [23] , [37] or near-infrared [38] region in the magnetic molecular and solid systems with chiral structures. Recently, another MCh dichroism has been reported for local d -electron excitation in a near-infrared region [39] and local spin excitation in a terahertz region [17] , [18] , where the magnetism assists the presence of the chirality in cooperation with the crystal symmetry. So far, the candidate materials for the MCh dichroism were restricted by the crystalline symmetry. On the other hand, the conical screw spin structure as investigated in this work gives rise to the chirality as well as the magnetization, irrespective of underlying lattice symmetry. Furthermore, the MCh dichroism demonstrated here is remarkably enhanced with the electromagnon resonance, namely, the strong ME coupling occurs in this resonance. In fact, the magnitude of the MCh dichroism ( Fig. 2c,e ), Δ κ ( ω )~0.3 or Δ κ ( ω )/ κ 0 ( ω )~1, are considerably high among the optical ME effects observed so far [17] , [18] , [22] , [23] , [37] , [38] , [39] . (Note that the normal term κ 0 ( ω )=( κ + ( ω )+ κ − ( ω ))/2 is derived from equation (2)). Therefore, the current result points to the advantage of the ME resonance derived from such a ubiquitous helical spin structure. The relation between the symmetry and the observed ME effect is worthy of consideration. The centrosymmetric crystallographic structure in the paramagnetic phase turns out to be a chiral lattice structure ( P 1 or P 2) in the screw spin phase through the spin–orbit interaction [40] , [41] . Since the screw axis along the magnetic modulation vector q m is the only symmetry element that can survive under application of the magnetic field ( H ex // q m // z) , some off-diagonal components ( α xy and α yx ) and diagonal components of the ME tensor should become nonzero. Although the diagonal element of the ME tensor contributes to the rotation of the polarization (gyrotropy), the negligibly small rotation is measured even in the maximum field strength (7 T) (see Methods). The observed result is in accord with for the spin–current mechanism, because this mechanism, producing the polarization ( ΔP ) perpendicular to the magnetization ( ΔM ) (see Fig. 1a ), contributes to the off-diagonal term of the ME tensor [21] . In contrast, the rotation of the light polarization by the natural optical activity driven by the diagonal term of the ME tensor has been reported for the local spin excitation on the Ba 2 CoGe 2 O 7 , in which the lattice symmetry and magnetism are cooperatively responsible for the chirality of matter [17] . The d–p orbital hybridization model including the local lattice geometry fully explains the natural optical activity as well as the MCh effect [17] . (Note that the first-order term of the d–p orbital hybridization model for delafossite structure such as CuFeO 2 is cancelled out [30] .) Therefore, critical difference of the optical response from this work suggests that the character of the optical ME effect strongly depends on their microscopic mechanism beyond simple estimation based on the symmetry. The ME effect implies the possible toroidal moment or its excitation, which stems from the spin orders or orbital currents in some cases [42] , [43] . The electromagnon observed here may be viewed as the excitation of the toroidal moment, because the toroidal moment is always anticipated under the presence of the cross-coupled ΔP ω and ΔM ω , that is, the dynamical ME effect [21] , [33] . In conclusion, we demonstrated the MCh effect on the electromagnon resonance for the conical screw spin structure in CuFe 1 −x Ga x O 2 ( x =0.035). The presence of the MCh dichroism was conclusively confirmed in terms of the control of the chirality (spin helicity) as well as the magnetization of the screw spins. Colossal MCh dichroism amounts to Δ κ ( ω )~0.3 or Δ κ ( ω )/ κ 0 ( ω )~1 on the electromagnon resonance. The optical ME effect demonstrated here is applicable to many frustrated magnetic systems as well as chiral magnets. This result opens a new door to the gigahertz and terahertz ME optics, such as isolator and filter devices, beyond the conventional optics. The use of the inverse MCh effect, for example, the photoproduction of magnetization, in terms of a high-field terahertz pulse will be also in sight as a possible extension of the phenomenon. Sample preparation and characterization Single crystal of CuFe 1 −x Ga x O 2 ( x =0.035) was grown by the floating-zone method. The size of the sample is 4 × 4 × 1 mm 3 with (110) plane. To manipulate the helicity- and q -domain of spin structure, the ME-cooling and magnetic q -flop procedures were employed as follows. Both magnetic field (7 T) along [100] and electric field (200 kV m −1 ) along [10] were applied in the cooling process. The electric field was turned off after the cooling. By rotating the magnetic field 60° from [100] to [110], the direction of the q was flopped from [100] to [110] due to the digital flop nature of the screw axis in this compound [29] . Terahertz optical spectroscopy Terahertz time-domain spectroscopy [44] was carried out under the magnetic field applied parallel to the light propagation direction (in the Faraday geometry) to determine the complex refractive index in a photon energy region from 0.8 to 2.5 meV. A femtosecond laser pulse was split into two paths to generate and detect the terahertz wave. The terahertz pulse was emitted from a bow-tie shape photoconductive antenna and detected by a dipole antenna. So as to estimate the contribution from Faraday rotation, the rotation angle of light polarization under the magnetic field was measured in crossed Nichol configuration. The rotation angle was confirmed to be <30 mrad T −1 for the 1-mm-thick sample, which least affects the κ ( ω ) value, at most by 0.02 at 7 T, in the quasi-linearly polarized analysis. The possible rotation derived from the natural optical activity, which would be expected under the presence of the spin-lattice coupling, was also examined. Even on the electromagnon resonance, the rotation angle was lower than our resolution limit, whose effect is 0.005 in κ ( ω ) at most. How to cite this article: Kibayashi, S. et al. Magnetochiral dichroism resonant with electromagnons in a helimagnet. Nat. Commun. 5:4583 doi: 10.1038/ncomms5583 (2014).